Interspecific introgression mediates adaptation to whole genome duplication Adaptive gene flow is a consequential phenomenon across all kingdoms. Although recognition is increasing, there is no study showing that bidirectional gene flow mediates adaptation at loci that manage core processes. We previously discovered concerted molecular changes among interacting members of the meiotic machinery controlling crossover number upon adaptation to whole-genome duplication (WGD) in Arabidopsis arenosa . Here we conduct a population genomic study to test the hypothesis that adaptation to WGD has been mediated by adaptive gene flow between A. arenosa and A. lyrata . We find that A. lyrata underwent WGD more recently than A. arenosa , suggesting that pre-adapted alleles have rescued nascent A. lyrata , but we also detect gene flow in the opposite direction at functionally interacting loci under the most extreme levels of selection. These data indicate that bidirectional gene flow allowed for survival after WGD, and that the merger of these species is greater than the sum of their parts. Whole-genome duplication (WGD) and hybridisation are key drivers of genomic novelty, promoting diversification in all kingdoms of life [1] , [2] , [3] . Recent progress in evolutionary genomics underscores the high frequency of WGD at both ancient and recent time scales [4] , and population genomic approaches reveal widespread evidence of gene flow between the most diverse species [5] , [6] . Both processes have therefore been associated with adaptive benefits. However, WGD and hybridisation are large-effect mutations, often leading to a host of genomic instabilities, including epigenetic shock, perturbed gene expression patterns and meiotic instability, with direct negative impacts on fertility. Perhaps the most challenging issue is the most immediate: that of stable meiotic chromosome segregation following WGD. How nascent polyploids establish meiotic stabilisation remains an unresolved question. The wild outcrossing members of the Arabidopsis genus have recently emerged as fruitful models for the study of genome stabilisation following WGD [7] . Arabidopsis arenosa is a largely biennial outcrossing relative of the model Arabidopsis thaliana , which forms distinct lineages of diploids and autotetraploids throughout Central Europe [8] , [9] , [10] , [11] . Initial resequencing of a handful of autotetraploid A. arenosa individuals suggested selective sweep signatures at genes involved in genome maintenance, including DNA repair, recombination and meiosis [12] . Later, a targeted resequencing effort focused on patterns of differentiation between diploid and autotetraploid A. arenosa , revealing evidence of highly localised selective sweeps directly overlapping eight loci whose gene products interact during prophase I of meiosis [13] . These eight loci physically and functionally interact to control crossover designation and interference, strongly implying that a modulation of crossover distribution was essential for polyploid establishment in A. arenosa [14] , [15] . Cytological evidence of a reduction in crossover numbers in the autotetraploids indicated that the selected alleles had an effect [13] . Similar to its sister species A. arenosa ( arenosa hereafter), Arabidopsis lyrata ( lyrata hereafter) also naturally occurs as diploids and tetraploids across its distribution range [8] , [16] , [17] , [18] . Although there is little evidence for gene flow among diploids of each species, there have been reports of gene flow between tetraploid arenosa and lyrata and, less pronounced, gene flow between diploids and tetraploids [8] , [19] , [20] . Here we investigate the molecular basis of parallel adaptation to WGD in lyrata compared with arenosa and the possibility of adaptive gene flow between the two species. Specifically, we ask (1) whether the same or different loci may be involved in adaptation to WGD in lyrata as we observed in arenosa ; and (2) whether these adaptations arose independently or via introgression from one species into the other. Using whole-genome sequence data from 92 individuals of lyrata , arenosa and outgroup species Arabidopsis croatica and Arabidopsis halleri , we first analyse population structure and demography, concentrating on assessing admixture and the degree and timing of population divergences. Then, to estimate the relative degree of adaptation to WGD across the ranges of lyrata and arenosa , we cytologically assess meiotic stability in key populations. Finally, after scanning the lyrata genomes for signatures of selective sweeps, we compare the most differentiated regions with those we previously found in arenosa [12] , [13] and test whether these selective sweep signatures overlap with fine-scale conspicuous introgression signals. Overall, our results reveal the molecular basis by which WGD has been stabilised in both species and indicate that WGD-facilitated hybridisation allowed for stabilisation of meiosis in nascent autotetraploids by highly specific, bidirectional adaptive gene flow. 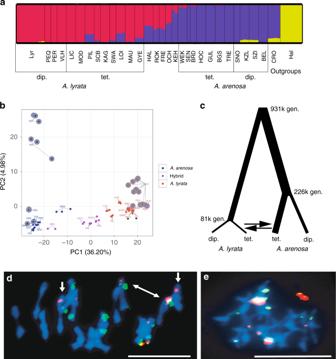Fig. 1 Ploidy-specific admixture and stable autotetraploid meiosis inA. lyrata.aA continuous range of admixture specifically in tetraploid populations demonstrated with STRUCTURE analysis of nuclear SNP data (32,256 LD-pruned, 4-fold degenerate SNPs). Populations (in three-letter code) and population groupings (ploidy, species) are displayed. Populations are described in (Supplementary Table1).bPCA shows individuals group on the main (PC1) axis by species and not by ploidy, with hybrid individuals located betweenA. lyrataandA. arenosasamples. We refer to all non-pure populations from the hybrid zone in the eastern Austrian Forealps as hybrids (see Supplementary Fig.1). Diploids are indicated by grey outline. Asterisks (*) are placed under theLettetraploid grouping; all otherA. lyratatetraploids (except the geographically divergent Pannonian GYE) are in theLwtgroup.cDemographic parameter estimates forA. lyrataandA. arenosapopulations. Line widths are proportional to estimates given in Supplementary Fig.2.d,eMetaphase I chromosome spreads of nuclei from two ROK plants hybridised with 5S rDNA (red) and 45S rDNA (green).dMI scored as stable as 16 individual bivalents are observed, even though there are bivalents with unequal probes (white arrows), suggesting non-homologous rearrangements.eMI scored as unstable as the majority of chromosomes are connected to each other. Chromosomes are stained with DAPI; bar = 10 µm. The source data underlying Fig.1d, eare provided as a Source Data file Population structure and broad-scale admixture To understand population and species relationships, we analysed the genomes of 92 individuals from ~30 populations of lyrata and arenosa throughout Central Europe along with outgroups, sequenced at a depth of ~15× per individual (Supplementary Table 1 and Supplementary Fig. 1 ). STRUCTURE and principal component analysis (PCA) showed a clear species-specific clustering for diploids, whereas tetraploids exhibited a gradient of relatedness between species (Fig. 1a, b ). Admixture was markedly lower in arenosa populations than in lyrata : consistently, all diploids tested (SNO, KZL, SZI, BEL) and tetraploids from the Western Carpathians (TRE), and most of the Alpine tetraploids (HOC, GUL, BGS) harboured essentially pure arenosa genomes (Fig. 1a ). Minimal admixture signal (<1%) with arenosa was detected in a few lyrata genomes, in particular the Austrian diploid (PEQ, PER, VLH), as well as the lyrata eastern tetraploid ( Let hereafter) populations (LIC, MOD) and the tetraploid KAG population (Fig. 1a ). Fig. 1 Ploidy-specific admixture and stable autotetraploid meiosis in A. lyrata . a A continuous range of admixture specifically in tetraploid populations demonstrated with STRUCTURE analysis of nuclear SNP data (32,256 LD-pruned, 4-fold degenerate SNPs). Populations (in three-letter code) and population groupings (ploidy, species) are displayed. Populations are described in (Supplementary Table 1 ). b PCA shows individuals group on the main (PC1) axis by species and not by ploidy, with hybrid individuals located between A. lyrata and A. arenosa samples. We refer to all non-pure populations from the hybrid zone in the eastern Austrian Forealps as hybrids (see Supplementary Fig. 1 ). Diploids are indicated by grey outline. Asterisks (*) are placed under the Let tetraploid grouping; all other A. lyrata tetraploids (except the geographically divergent Pannonian GYE) are in the Lwt group. c Demographic parameter estimates for A. lyrata and A. arenosa populations. Line widths are proportional to estimates given in Supplementary Fig. 2 . d , e Metaphase I chromosome spreads of nuclei from two ROK plants hybridised with 5S rDNA (red) and 45S rDNA (green). d MI scored as stable as 16 individual bivalents are observed, even though there are bivalents with unequal probes (white arrows), suggesting non-homologous rearrangements. e MI scored as unstable as the majority of chromosomes are connected to each other. Chromosomes are stained with DAPI; bar = 10 µm. The source data underlying Fig. 1d, e are provided as a Source Data file Full size image In contrast, many other lyrata populations exhibited substantial admixture signals with arenosa , varying drastically in degree (Fig. 1a ). Several tetraploid lyrata populations from the Wachau (SCB, SWA, MAU) displayed only slight admixture with arenosa and populations at the Wachau margin (PIL, LOI) showed stronger admixture, probably due to the increased proximity to the Hercynian and Alpine arenosa lineages [21] . Compared with the Wachau, where lyrata occurs on the slopes and hilltops along the Danube river surrounded by arenosa populations outside of the valley, there is a classical hybrid zone in the eastern Austrian Forealps: the parental species are found at the two poles of the zone (diploid and tetraploid lyrata in the Wienerwald, tetraploid arenosa at higher altitudes to the west and the hybrids between; Supplementary Fig. 1 ). Populations HAL, ROK, FRE, OCH and KEH are heavily admixed, with KEH appearing more arenosa -like, and ROK and FRE being slightly more lyrata -like compared with the others (Fig. 1a ). Again, proximity of the hybrids to the donor species corresponded with increased admixture. The Hungarian tetraploid lyrata population GYE also exhibited admixture signal, suggesting that gene flow between lyrata and arenosa is not restricted to the Austrian Forealps. PCA was consistent with STRUCTURE findings, with PC1 dividing samples by species (explaining >36% of the variance; Fig. 1b ). The second axis (<5% of the variance) separated KZL and SZI from the other diploid arenosa populations. These are representatives of the Pannonian lineage, which is the oldest and most distinct diploid arenosa lineage [21] . Overall, our results are consistent with previous descriptions of introgression between lyrata and arenosa in Austria that were based on smaller marker sets and different sampling schemes [8] , [22] . We estimated the population split time without migration between lyrata and arenosa at 931,000 (931k) generations ago using fastsimcoal2 [23] (Fig. 1c , Supplementary Figs. 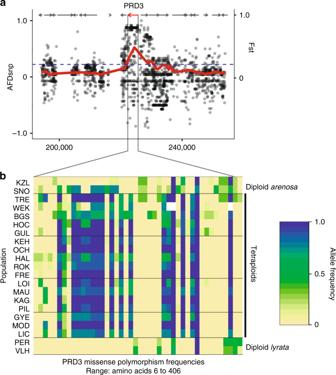Fig. 2 Selective sweeps and missense polymorphism frequencies by population.aSelective sweep example inPRD3, a gene involved in meiotic double strand break formation.X-axis gives chromosome 1 position in base pairs. LeftY-axis gives allele frequency differences between diploid and tetraploidA. lyrataand at single-nucleotide polymorphisms (dots). RightY-axis (and red line) gives local Fst. Arrows indicate gene models. Red arrow indicates selective sweep candidate with localised differentiation. The dotted line gives the 99th percentile of genome-wide Fst values.bZoom-in onPRD3coding changes. Heatmap represents allele frequencies of missense polymorphisms. Frequencies 0–100% follow yellow to green, to blue. Derived diploidA. arenosa-specific missense polymorphisms are driven to high frequency in the tetraploids, whereas diploidA. lyrataalleles are absent, implicating diploidA. arenosaorigin to this selected allele in the tetraploids 2 and 3 , and Supplementary Table 2 ). This translates to ~2 million years ago (mya), given an average generation time of 2 years, which would coincide with the onset of Pleistocene climate oscillations. This estimate lies within the range of age estimates for this split from ref. [24] with 1.3 mya and from ref. [25] with 8.2 mya, and ref. [22] . We estimated the age of WGDs at 81k generations ago for lyrata (~160,000 years ago) and 226k generations ago for arenosa (~450,000 years ago), which approximately mark periods of glacial maxima [26] . Noting this, we next asked if either species experienced substantial historical bottlenecks. Using pairwise sequentially Markovian coalescent (PSMC) model [27] we could not reach ages as ancient as 130–300 kya (Supplementary Fig. 4 ), because the recombinant blocks that PSMC measures are too short in these diverse outcrossing species to estimate ancient population histories. Our analysis indicated that diploid lyrata had a peak effective population size ( Ne ) ~25 kya (PER, VHL) and ~20 kya (PEQ), whereas diploid Dinaric arenosa (BEL) peaked earlier, at ~30 kya. Interestingly, diploid Western Carpathian arenosa SNO, the population that founded several widespread autotetraploid lineages [9] , gave a strong signal of continuous expansion. These results suggest that diploid lyrata and partly arenosa underwent a bottleneck after the last glacial maximum 30–19 kya. PSMC does not accommodate autotetraploid data, but using fastsimcoal2 we detected a strong bottleneck at WGD for lyrata and none for arenosa (Supplementary Fig. 2 ). We next assayed for patterns of gene flow using coalescent modelling with fastsimcoal2 . Due to model overfitting when using more than two migration edges, we chose the model retaining only two migration edges with the highest support: interspecific gene flow from tetraploid arenosa to tetraploid lyrata (0.1 alleles/generation) and lyrata to arenosa gene flow at the same level (0.1 alleles/generation) (Fig. 1c , Supplementary Figs. 2 and 3 , and Supplementary Table 2 ). These results indicate equal amounts of bidirectional gene flow specifically among the tetraploids of both species. Stabilisation of lyrata meiosis following WGD Given the very low abundance of lyrata tetraploids compared with tetraploid arenosa in nature, we assayed whether these tetraploids were indeed meiotically stable. Cytological analysis indicated that in fact lyrata tetraploids exhibit similar levels of meiotic stability as arenosa tetraploids, as evidenced by relative percentages of stable rod and ring bivalents (Fig. 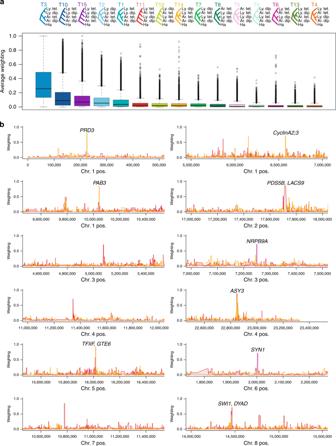Fig. 3 Highly specific introgression events across species boundaries.aTopologies fromTwisstanalysis ofLwt: Although topology 3 is the dominant species tree, topologies 11, 14 and 6 indicate localised gene flow between tetraploids. Box plots give relative weightings of all topologies across the genomes analysed. It is noteworthy that the extreme outliers concentrate specifically on the introgression-indicative topologies 11, 14 and 6. The bold line indicates the median. The box spans the first and third quartiles, and the whiskers extend to the most extreme point within 1.5 times the interquartile range from the box. Source data are provided as a Source Data file.bIntrogression events revealed byTwisstanalysis are highly localised at loci encoding genes controlling meiosis, endopolyploidy, and transcriptional control. All gene-coding loci under a given narrow peak are labelled; many of the indicated loci are divergence scan outliers in both theLetandLwtdivergence scans in addition to being Twisst outliers. The genome-wide dominant topology 3 weightings are omitted inbfor clarity. The colours inbcorrespond to topologies 11, 14 and 6 ina. The weighting quantifies the extent to which each 50 SNP window tree matches a given topology, accounting for the fact that each taxon is represented my multiple individuals that each have 2 (for diploids) or 4 (for tetraploids) tips in the tree. A weighting of 1 indicates that all individuals cluster in the same way, such that all possible subtrees match the same topology. Weightings >0 but <1 indicate that different subtrees match different topologies. Source data are provided as a Source Data file 1d and Supplementary Table 3 ) vs. less stable multivalents (Fig. 1e and Supplementary Table 3 ). We were surprised to observe among both species that meiotic stability segregates within populations, typically ranging from <20 to >60% stable metaphase I cells per plant with extremes observed in KAG (0–98%) and consistently higher levels (>80%) in the arenosa populations. Meiotic stability was also variable within the tetraploid arenosa population TBG, which was the population used by Yant et al. [13] to cytologically assess meiotic stability. A much higher number of chromosome spreads on more individuals and populations in the present study indicates that meiosis is not universally stable among autotetraploids across these populations. Overall, these results indicate that meiotic stability is broadly segregating within tetraploid populations of both species. Selective sweep signatures in lyrata To gain insight into the processes underlying adaptation to WGD in lyrata tetraploids, we performed a population-based genome scan for selection. We quantified differentiation between lyrata ploidies by calculating d XY [28] , Fst [29] and Rho [30] in adjacent windows along the genome between diploids and tetraploids. Fst is influenced by within-population diversity and lacks sensitivity in cases of low differentiation. Therefore, we used additional differentiation metrics. d XY does not take within-population diversity into account, whereas Rho is a divergence measure that is independent of ploidy level and double reduction in autopolyploids. We focused on the non-admixed lyrata tetraploid populations LIC and MOD ( lyrata eastern tetraploids; Let ), which by STRUCTURE and PCA analyses exhibited the lowest levels of admixture (Fig. 1a ) and clustered with lyrata diploids, distant from the arenosa tetraploids or the broadly admixed lyrata tetraploids (Fig. 1b ). Overall, genome-wide differentiation levels between lyrata diploids and the tetraploids indicate shallow divergence between all groups (with mean Rho in the most differentiated contrast between ploidies = 0.19; Table 1 and Supplementary Table 4 for additional population contrasts), consistent with our previous studies in arenosa [12] , [13] , [21] , [31] . Table 1 Genome-wide differentiation between A. lyrata diploids and tetraploids, and between tetraploid lineages grouped by biogeography Full size table To identify the most robust signals of selection in the tetraploid lyrata populations, we performed genome scans on two different lyrata tetraploid population groups and then focussed on the genes that were repeatedly in the extreme 1% outlier windows in both contrasts. This identified 196 genes (0.6% of gene-coding loci in the genome; Supplementary Dataset 1 ). First, contrasting the lyrata diploids and the Let tetraploids, we partitioned the genome into gene-sized windows and identified outliers for allele frequency differences (AFDs), d XY , Fst, Rho and the number of fixed differences. Although the comparison of the most pure lyrata tetraploid populations, represented by the Let group, to lyrata diploids is the most stringent test of which loci are under selection in a purely lyrata genomic context, we extended our tetraploid lyrata sampling to populations from the Wachau, which frequently showed admixture with arenosa ( lyrata Wachau tetraploids, Lwt hereafter: PIL, SCB, KAG, SWA, LOI and MAU; GYE was excluded due to distant geographic grouping in Pannonia). As the Let and part of the Lwt populations grow in contrasting edaphic conditions ( Let on limestone, Lwt on siliceous bedrock), we used this approach to maximise our chances of capturing differentiation specifically related to ploidy and not local adaptation. In addition, we observed that differentiation between these two tetraploid lyrata groups is stronger than differentiation between the tetraploid arenosa lineages studied here (Table 1 ), suggesting that there is stronger genetic structure within lyrata than arenosa , as was observed by ref. [32] , and supporting a degree of independence between the Let and Lwt divergence scans. Gene Ontology (GO) enrichment analysis of these 196 genes identified significant overrepresentations in categories related to meiotic and homologous chromosome segregation, but also diverse processes including epidermal cell differentiation, trichoblast maturation, root hair cell and epidermal differentiation, root hair cell development and elongation, and others such as indole-containing compound metabolic process and mRNA catabolic process (Supplementary Fig. 5 and Supplementary Dataset 2 ). These results indicate that evolutionary change may occur throughout a broad array of processes during adaptation to WGD, beyond meiotic chromosome segregation. Comparing this set of outliers to those found under selection upon WGD in arenosa [13] , 20 gene-coding loci exhibited the highest levels of differentiation in both studies (Table 2 ). These included those meiosis-related loci reported above ( PRD3 , ASY1 , ASY3 and SYN1 ), as well as the endopolyploidy genes CYCA2;3 and MEE22 , and the global transcriptional regulator TFIIF , among others. We observed selective sweep signatures at the majority (6/11) of coding loci of known function that were found as the very top outliers in arenosa (0.5% outliers for all three metrics used in that study) having primary functions of mediating meiosis, endopolyploidy and transcription. In particular, outlier loci participating in meiotic crossover formation, including ASY1 , ASY3 , PDS5-like , PRD3 , and SYN1 exhibited tight peaks of divergence directly over single gene-coding loci (an example is given in Fig. 2 ), a divergence signal we have broadly seen in this system [13] , [21] , [31] . In addition, the meiosis loci important for crossover formation reported by Yant et al. [13] ZYP1b and PDS5 were outliers in the Lwt contrast. The paralog ZYP1b was differentiated in the Let group also, but was not among the 1% top outliers; PDS5 showed no differentiation between the Let and lyrata diploids. SMC3 , a top outlier in arenosa , showed only moderate differentiation in the Lwt and no differentiation in the Let scan. Taking this most restrictive list representing the overlap of three genome scans, GO enrichment analysis identified significant overrepresentations only in categories related to meiotic chromosome segregation (Supplementary Dataset 3 ). These results further support the notion that these same loci were under the highest levels of selection following the more recent WGD event in lyrata as were under selection following the independent, earlier WGD (Fig. 1c ) in arenosa . Table 2 Overlap list of the top 1% outliers from the genome scans Full size table Fig. 2 Selective sweeps and missense polymorphism frequencies by population. a Selective sweep example in PRD3 , a gene involved in meiotic double strand break formation. X -axis gives chromosome 1 position in base pairs. Left Y -axis gives allele frequency differences between diploid and tetraploid A. lyrata and at single-nucleotide polymorphisms (dots). Right Y -axis (and red line) gives local Fst. Arrows indicate gene models. Red arrow indicates selective sweep candidate with localised differentiation. The dotted line gives the 99th percentile of genome-wide Fst values. b Zoom-in on PRD3 coding changes. Heatmap represents allele frequencies of missense polymorphisms. Frequencies 0–100% follow yellow to green, to blue. Derived diploid A. arenosa -specific missense polymorphisms are driven to high frequency in the tetraploids, whereas diploid A. lyrata alleles are absent, implicating diploid A. arenosa origin to this selected allele in the tetraploids Full size image Apart from loci encoding meiosis-related genes, we detected extreme differentiation at loci belonging to other functional categories clearly related to the challenges attendant to WGD, including loci involved in endoreduplication and transcriptional regulation: CYCA2;3 , PAB3 , NAB , TFIIF and GTE6 . WGD increases the ploidy of all cells, whereas endopolyploidy occurs in single cells during their differentiation, and this cell- and tissue-specific ploidy variation is important in plant development [33] , [34] , [35] . Thus, given the instantly doubled organism-wide nuclear content following WGD, we postulate that the degree of endopolyploidy would be modulated in response, with accumulating support for this notion [36] , [37] , [38] . Our findings bolster the idea that there may be a link between organism-wide polyploidization, and that of single cells within an organism. Research about the effect of WGD-induced dosage responses of the transcriptome is still in its infancy [3] , [39] and emerging studies on allopolyploids support incomplete dosage compensation. Highly specific introgression at sweep genes Finally, we sought to confirm whether the strong observed signals of selective sweep were the products of localised interspecific introgression. To confirm candidate introgressed regions at high resolution, we used Twisst [40] , performing two independent analyses, with either Let or Lwt representing tetraploid lyrata . The consensus species phylogeny, topology 3, represented the overwhelmingly dominant genome-wide topology (Fig. 3a ). Topologies consistent with introgression (6, 11 and 14, which group tetraploids of the two species together) all had comparatively low values, but also showed multiple narrow peaks across the genome. Twelve peaks had weightings >0.7 and nine of these overlapped with our divergence scan outliers (Fig. 3b and Supplementary Dataset 4 ). Similarly, 61 had a weighting >0.5 and 21 (34%) of these overlapped with gene-coding loci that were positive in both the Let and Lwt divergence scans (Fig. 3b and Supplementary Dataset 4 ). This degree of overlap of the loci found under selection in our genome scans is dramatically greater than expected by chance (0.6%), which we confirmed by performing permutation tests (Supplementary Fig. 6 ). By contrast to the introgression-indicative topologies, those consistent with incomplete lineage sorting (ILS) alone (7, 8, 9, 12 and 13, which group diploid arenosa with tetraploid lyrata or vice versa) were low genome-wide with only two peaks reaching above 0.5 (Fig. 3a ). Fig. 3 Highly specific introgression events across species boundaries. a Topologies from Twisst analysis of Lwt : Although topology 3 is the dominant species tree, topologies 11, 14 and 6 indicate localised gene flow between tetraploids. Box plots give relative weightings of all topologies across the genomes analysed. It is noteworthy that the extreme outliers concentrate specifically on the introgression-indicative topologies 11, 14 and 6. The bold line indicates the median. The box spans the first and third quartiles, and the whiskers extend to the most extreme point within 1.5 times the interquartile range from the box. Source data are provided as a Source Data file. b Introgression events revealed by Twisst analysis are highly localised at loci encoding genes controlling meiosis, endopolyploidy, and transcriptional control. All gene-coding loci under a given narrow peak are labelled; many of the indicated loci are divergence scan outliers in both the Let and Lwt divergence scans in addition to being Twisst outliers. The genome-wide dominant topology 3 weightings are omitted in b for clarity. The colours in b correspond to topologies 11, 14 and 6 in a . The weighting quantifies the extent to which each 50 SNP window tree matches a given topology, accounting for the fact that each taxon is represented my multiple individuals that each have 2 (for diploids) or 4 (for tetraploids) tips in the tree. A weighting of 1 indicates that all individuals cluster in the same way, such that all possible subtrees match the same topology. Weightings >0 but <1 indicate that different subtrees match different topologies. Source data are provided as a Source Data file Full size image Similar to the divergence outlier windows, Twisst -positive windows were narrow, which might be an indication that genomic differentiation following divergence between lyrata and arenosa is advanced and introgression occurred fairly deep in the past, similar to the numerous narrow genomic regions of introgression in the case of gene flow between Populus alba and Populus tremula [41] . However, we have recently estimated linkage disequilibrium (LD) in this system [21] , finding a very rapid reduction specifically in the autotetraploid cytotype (50% lower mean correlations at 1 kb distance), suggesting that tight introgression signals may be formed rapidly in this system. Although sharing of adaptive alleles between tetraploid populations can also be explained by ILS, the symmetrical design of our study allows us to reject ILS in most cases. Under ILS, we expect two divergent alleles to have existed in the ancestor of both species, which would lead to topology 6 after sorting of these alleles into diploids and tetraploids, respectively. Of the top 12 Twisst peaks, only one represents topology 6. The others represent topologies 11 and 14, in which the tetraploid alleles are nested within the diploids, implying that they arose after speciation and subsequently introgressed (Fig. 3a ). A slight majority of these loci with introgression signal appear to have a lyrata origin (30/53 Twisst peaks), but among those with the highest levels of selection in Lwt , Let , and arenosa , a majority (11/16 where direction can be inferred) harbour evidence of an arenosa origin (Supplementary Dataset 4 ). GO enrichment analysis of the gene-coding loci in the windows where direction could be inferred found only enrichment for categories related to meiosis (Supplementary Datasets 5 and 6 ). Taking these results together, we observe that four meiosis-related loci were outliers in all Twisst and divergence scans: PRD3 , ASY3 , SYN1 and DYAD , and four did not show a signal in both Twisst analyses as well as both divergence scans: ASY1 , ZYP1a , ZYP1b and PDS5 . Given that arenosa is the much older tetraploid (2.5 times as ancient as lyrata ; Fig. 1c ) and is much more widespread, we hypothesise that arenosa -sourced alleles were under selection for stable polyploid meiosis longer, providing pre-adapted alleles to the nascent lyrata tetraploid, although this hypothesis needs to be functionally tested in dedicated studies. Introgression of optimised alleles from an older to a younger species has been indicated for high-altitude adaptive alleles from Denisovans and Tibetan Homo sapiens [42] . Taking PRD3 as a clear example (Fig. 2b ), derived arenosa -specific missense polymorphisms in the diploid population SNO are driven to high frequency in the tetraploids of both species, whereas diploid lyrata alleles are absent, strongly implicating a specific diploid arenosa origin in this case. At the same time, we detect specific signals of gene flow from lyrata into arenosa . In addition to meiosis-related genes, we see introgression signal at the endopolyploidy gene CYCA2;3 and the global transcriptional regulator TFIIF , but very few other loci exhibit both persistent signatures of extreme selection as well as introgression (Supplementary Datasets 3 and 4 ). Our findings suggest that introgression of particular alleles of meiosis-related genes might stabilise polyploid meiosis, with the less effective alleles of one species being replaced by introgression of alleles from orthologous loci in the other tetraploid. Introgression of alleles optimised for adaptation to WGD could be especially beneficial in hybrid zones such as this one, which spans a climatic gradient from a warmer, Pannonian climate at its eastern margin to harsher conditions in the eastern Alps. Meiosis is a temperature-sensitive process [15] and we hypothesise substantial levels of meiosis-related allele–environment associations with variable temperature. Allele–environment associations with climatic variables across a hybrid zone have been observed in spruce [43] . For these newly formed tetraploids, WGD appears to be both a blessing and a curse. Although WGD appears to have opened up access to the allelic diversity of a sister species, as well as provided population genomic benefits [21] , it also presents new challenges to the establishment of optimal allelic combinations. As the gene products at the meiotic loci under the most extreme selection across this hybrid zone functionally and physically interact, we expect that efficient evolved polyploid meiosis requires the harmonious interactions of multiple selected, introgressed alleles in concert. However, relatively high levels of residual masking of genetic load in autotetraploids [21] , [44] will tend to extend the duration that deleterious alleles segregate in populations, with negative phenotypic consequences. This is consistent with our observation that polyploid meiosis exhibits wide degrees of within-population variability in stability. This observed diversity suggests that the optimal combination of meiosis alleles is yet segregating, which may also be the result of the recent age of these WGDs. Dedicated molecular investigation of whether the measured within-population meiotic stability is associated with particular allele combinations is the focus of ongoing functional analyses. In this study, we investigated the population genetic basis of adaptation to WGD in congeners that, due to an endosperm-based postzygotic barrier [20] , hybridise only as tetraploids. We found that many of the same loci exhibit the most conspicuous signatures of selective sweep in lyrata following WGD that we observed in arenosa , and further, that the strongest signals of interspecific introgression occur precisely at many of these same loci. Using whole-genome sequence data from 30 populations, we probed complex population structure and patterns of gene flow. Interestingly, we observed cytologically that the degree of meiotic stability varied dramatically, even within populations of both species, suggesting that stability has not been completely established, or that other, perhaps epigenetic or environmental factors influence meiotic stability in still unknown ways. At the same time, populations exhibited admixture signals that contrast dramatically in degree, indicating a complex introgression landscape. We present evidence that the molecular basis by which WGD was stabilised in lyrata and arenosa is shared. Our data further suggest that WGD-facilitated hybridisation allowed for stabilisation of meiosis in nascent autotetraploids by specific, bidirectional adaptive gene flow, tightly overlapping loci known to be essential for processes that are impacted by WGD: meiotic stability, endopolyploidy, and transcription, and others. It is curious that the very process that rescues fitness in these species, hybridisation, is potentiated by the same phenomenon to which the resultant adaptive gene flow responds: WGD. Sample design and sequencing Individual plants were collected from field sites across Central Europe (Supplementary Fig. 1 ). Cytotypes were determined by flow cytometry from these populations in ref. [8] and ref. [21] , no triploids have been detected in these populations, nor have we found any evidence in the flow cytometry or cytology data that any of these populations consist of mixed-ploidy subpopulations. Central European tetraploid lyrata has its largest distribution in eastern Austria, in two biogeographic regions: the Wienerwald ( lyrata eastern tetraploids/ Let hereafter; LIC, MOD), and the Wachau ( lyrata Wachau tetraploids/ Lwt hereafter; PIL, SCB, KAG, SWA, LOI, MAU). We found an additional tetraploid lyrata population in Hungary (GYE) and included it in this study. Diploid lyrata populations were chosen from the Wienerwald (PEQ, PER, VLH), which are the geographically closest diploid populations to the Let and Lwt , and therefore likely serve as source populations. For arenosa , representative populations of tetraploids from the Hercynian (WEK, SEN, BRD) and Alpine lineages (HOC, GUL, BGS) were selected, as well as additional arenosa populations from the Western Carpathians (diploid: SNO; tetraploid: TRE), which is the centre of arenosa genetic diversity and the region of origin of the tetraploid cytotype [9] . For breadth, we selected several more diploid arenosa populations from the Pannonian (KZL, SZI) and Dinaric (BEL) lineages, as well as the following populations from the hybrid zone in the eastern Austrian Forealps: HAL, ROK, FRE, OCH and KEH. To complement our sampling with diploid lyrata from across its entire distribution range, we selected samples from the Hercynian (SRR2040791, SRR2040804), arctic-Eurasian (SRR2040796, SRR2040798, SRR2040805) and arctic-North American lineages (DRR054584, SRR2040769, SRR2040770, SRR2040789). A. croatica (CRO) and A. halleri (SRR2040780, SRR2040782, SRR2040783, SRR2040784, SRR2040785, SRR2040786, SRR2040787) were included as outgroups [32] . The majority of lyrata and hybrid samples were collected as seeds, cultivated and flash-frozen prior to DNA extraction, whereas samples for three populations (LIC, MOD, HAL) were collected and silica-dried. Silica-dried material from GYE was obtained from Marek Šlenker and Karol Marhold. Arenosa samples were collected and sequenced as part of a different study [21] . In addition, 16 accessions were downloaded from the NCBI Sequence Read Archive (SRA), bringing the total sample number to 92 (Supplementary Table 1 ). DNA of the lyrata and hybrid samples was extracted and purified from frozen or silica-dried leaf and/or flower tissue using the Epicentre MasterPure DNA extraction kit. DNA concentration measurements were performed with the Qubit 3.0 fluorometer (Invitrogen/Life Technologies, Carlsbad, California, USA). Genomic libraries for sequencing were prepared using the Illumina TRUSeq PCR-free library kit with 500 ng to 1 μg extracted DNA as input. We multiplexed libraries based on the Qubit concentrations, and those multiplexed mixes were run on an initial quantification lane. According to the yields for each sample, loading of the same multiplex mix on several lanes was increased to achieve a minimum of 15× coverage. Samples that had less than our target coverage were remixed and run on additional lanes. Libraries were sequenced as 125 bp paired-end reads on a HiSeq2000 by the Harvard University Bauer Core Facility (Cambridge, MA, USA). Data preparation and genotyping Newly generated sequencing data and SRA accessions were processed together from raw fastq reads. We first used Cutadapt [45] to identify and remove adapter sequences with a minimum read length of 25 bp and a maximum error rate of 0.15. We then quality trimmed reads using TRIMMOMATIC [46] (LEADING:10 TRAILING:10 SLIDINGWINDOW:4:15 MINLEN:50). Samples sequenced on several lanes were then concatenated using custom scripts. Reads were deduplicated using MarkDuplicates in picard v.1.103. Broadinst and readgroup names were adjusted utilising AddorReplaceReadGroups within the picard package. Reads were then mapped to the North American lyrata reference genome (v.2 [47] ) using bwa-mem in the default paired-end mode [48] . Indels were realigned using the Genome Analysis Toolkit (GATK) IndelRealigner. Prior to variant discovery, we excluded individuals that had fewer than 40% of bases <8× coverage (assessed via GATK’s DepthOfCoverage with the restriction to a minimum base quality of 25 and a minimum mapping quality of 25). Our final dataset for analysis contained 92 individuals. Variant calling was performed using the GATK HaplotypeCaller (--min_base_quality_score 25 --min_mapping_quality_score 25 -rf DuplicateRead -rf BadMate -rf BadCigar -ERC BP_RESOLUTION -variant_index_type LINEAR -variant_index_parameter 128000 --pcr_indel_model NONE), followed by GenotypeGVCFs for genotyping. For each BAM file, HaplotypeCaller was run in parallel for each scaffold with ploidy specified accordingly and retaining all sites (variant and non-variant). We combined the single-sample GVCF output from HaplotypeCaller to multisample GVCFs and then ran GenotypeGVCFs to jointly genotype these GVCFs, which greatly aids in distinguishing rare variants from sequencing errors. Using GATK’s SelectVariants, we first excluded all indel and mixed sites and restricted the remaining variant sites to be biallelic. Additional quality filtering was performed using the GATK VariantFiltration tool (QD < 2, MQ < 40.00, FS > 60.0, SOR > 4.0, MQRankSum < − 8.0, ReadPosRankSum < − 8.0, DP < 8). Then we masked sites that had excess read depth, which we defined as 1.6× the second mode (with the first mode being heterozygous deletions or mismapping) of the read depth distribution. Population structure All analyses dedicated to reveal population structure and demography were based on putatively neutral fourfold degenerate (4dg) single-nucleotide polymorphisms (SNPs) only. We used the 4dg filter generated for arenosa from ref. [9] . After quality filtering, these analyses were based on a genome-wide dataset consisting of 4,380,806 4dg SNPs, allowing for a maximum of 10% missing alleles per site (1.2% missing data) at a 5× coverage minimum for a given individual sample. Although we expected fastSTRUCTURE [49] to be superior in recognising admixture compared with STRUCTURE [50] , running fastSTRUCTURE on our dataset resulted in poor performance, in that the result did not coincide with the STRUCTURE results or other analysis. This misbehaviour was probably due to the inclusion of polyploid data, as fastSTRUCTURE does not accommodate polyploid genotypes. We had randomly subsampled two alleles per each tetraploid site, similar to ref. [32] , using a custom script. However, evidently such a subsampling strategy dissolves the fine-scale differences in admixture between populations at this scale. Hence, STRUCTURE was preferred, and was run on all samples and both ploidies. As STRUCTURE accepts only uniform ploidy as input, with one row per each ploidy, we added two rows of missing data for our diploid samples, making them pseudo-tetraploid. In addition, input data were LD-pruned and singletons removed using custom scripts. Window size was set to 500 with a distance of 1000 between windows, allowing for 10% missing data, which resulted in a dataset of 32,256 SNPs genome wide. We performed ten pruning replicates using the admixture model with uncorrelated allele frequencies, and then ran each for K -values 2–10 with a burn-in period of 50,000 and 500,000 Markov Chain Monte Carlo (MCMC) replicates. We conducted PCA using the glPca function in the adegenet R package [51] . Demographic parameters and reconstruction of gene flow We next performed demographic analyses with fastsimcoal2 [23] on 4dg sites. A minimum of two individuals per each population was required. Custom python scripts (FSC2input.py at https://github.com/pmonnahan/ScanTools/ ) were used to obtain the multi-dimensional allele frequency (DSFS) spectrum as well as bootstrap replicates of the DSFS for confidence interval estimation. For the bootstrap replicates, the genome was divided into 50 kb segments and segments were resampled with replacement until recreating a DSFS of equivalent size as the genome. Ultimately, we aimed to estimate demographic parameters and confidence intervals for a four-population tree corresponding to diploid and tetraploid lyrata and arenosa . For computational efficiency, three-population trees were initially used to establish the presence/absence of migration edges by comparing models with a single migration edge to a null model with no migration. Additional migration edges would then be added and compared with the initial simple model. For each model, 50 replicates were performed and values kept for the replicate with the highest likelihood. For each replicate, we allowed for 40 optimisation cycles and 100,000 simulations in each step of each cycle for estimation of the expected side frequency spectrum. Although the above process identified the key migration edges, it resulted in a four-population tree that was overly complex; the exercise suggested six migration edges in total (Supplementary Fig. 3 ). Overfitting was evidenced by highly imprecise and nonsensical estimates for a subset of parameters (Supplementary Table 2 ). For example, the ancestral population size for lyrata was estimated to be greater than 5 million with individual replicate estimates ranging from <100,000 to over 10 million. Estimates for population fusion times were also drastically greater than observed in previous three-population trees. We therefore opted for a simpler model, retaining only the two migration edges with the highest support: bidirectional migration between tetraploids. Parameter estimates for each of the 100 bootstrap replicates were obtained using the scheme described above, and 95% confidence intervals were calculated using the 2.5th and 97.5th percentiles of the resulting distribution of each parameter. Changes in effective population size over time PSMC model v.0.6.4 was used to infer changes in effective population size ( Ne ) through time using information from whole-genome sequences of lyrata and arenosa diploids [27] . We generated plots of the most deeply sequenced representative of each of the diploid lyrata and arenosa populations, with the exception of distinct arenosa KZL and SZI. A consensus fastq sequence was created using samtools v.1.2 and bcftools v.1.2 using samtools mpileup -C50 -Q 30 -q 30 with the lyrata v.2 genome as the reference. The reference was masked at all sites at which read depth was more than twice the average read depth across the genome. Samtools mpileup was followed with bcftools call -c and vcfutils.pl vcf2fq -d 5 -D 34 -Q 30 to create a fastq reference file. Using PSMC, this was changed to a format that was required with PSMC by fq2psmcfa -q20, and psmc was run with parameters psmc -N25 -t15 -r5 -p “4 + 25*2 + 4 + 6” and psmc_plot.pl -R -g 2 -u 3.7e-8 to get a text file that could be plotted with R . We used the mutation rate estimate μ = 3.7 × 10 −8 [9] and a generation time of 2 years for both species, as arenosa is mainly biennial, and we estimate that lyrata generates the highest number of propagules in its second year after germination (R.S., personal observation). Cytological assessment of meiotic stability Individual tetraploid lyrata and arenosa plants were germinated in 7 cm pots with Levington® Advance Seed and Modular Compost Plus Sand soil with 16 h light/8 h dark cycles at 20 °C constant temperature. Once rosettes had formed, plants were vernalised for six weeks with 8 h light (6 °C)/16 h dark (4 °C) cycles. Plants were then grown in 16 h light (13 °C)/8 h dark (6 °C) cycles to encourage flowering. Buds were collected, fixed and anthers dissected for basic cytology as described in [52] except that 50 mg (30 Gelatine Digestive Units) Zygest® Bromelain were added to the enzyme mixture, and incubation time was increased to 75 min. The prepared slides were stained and mounted with 7 µl 4′,6-diamidino-2-phenylindole (DAPI) in Vectashield (Vector Lab) and metaphase I chromosomes visualised using a Nikon 90i Eclipse fluorescent microscope with NIS Elements software. Chromosome spreads with all rod and/or ring bivalents were scored as stable meiosis (Fig. 1d ), whereas multivalents with multiple chiasmata were scored as unstable meiosis (Fig. 1e ). FISH was performed as in [52] , except 62 °C was used as the chromosome denaturing temperature. The 5S rDNA probe was generated by directly incorporating biotin into a PCR product (Jenna Biosciences) using primers 5SF 5′-AACCGAAATTGCGTGCATAG-3′ and 5SR 5′-AAACGGGAGGTGAGACGAG-3′ with Mimulus guttatus cloned genomic DNA that shares 96% nucleotide identity with A. lyrata in this region and the 45S pTa71 clone (Gerlach and Bedbrook, 1979) by nick translation with digoxigenin (Jenna Biosciences). Streptavidin Dylight 594 and anti-digoxigenin Dylight 488 (Vector laboratories) were used as secondary fluorophores. Chromosomes were stained with DAPI in Vectashield (Vector Laboratories). Differentiation scans for signatures of selective sweeps We grouped populations by ploidy level, species or hybrid affiliation, and affiliation to a biogeographic region in case of tetraploid lyrata . We calculated the following metrics in adjacent nonoverlapping genomic windows: AFD, d XY , Fst [53] , Rho [30] and the number of fixed differences between the lyrata diploids and the two lyrata tetraploid groups ( Let and Lwt ). We identified selective sweep candidates as the 1% outliers of the empirical distribution for each metric. To maximise our chances of capturing differentiation truly related to ploidy and not local adaptation, we selected the overlap between these two independent scans wherein the tetraploids contrast by edaphic (soil) preference and then focused on outliers that were identified in a highly stringent genome scanning approach in arenosa [13] . To obtain insight into differentiation between population groups, AFD, d XY , Fst, Rho, and the number of fixed differences were calculated for additional populations. Arenosa populations were grouped by lineage, as identified in refs. [9] , [21] , as arenosa Hercynian tetraploids ( Aht ) and arenosa Alpine tetraploids ( Aat ), which also corresponds to biogeographic groupings. GO enrichment analysis We performed gene function enrichment tests for each contrast using the CLUEGO app version 2.5.4 in CYTOSCAPE version 3.7.2 using GO information associated with orthologous A. thaliana gene identifiers. We retained levels 3-8 for biological process (Benjamini-Hochberg correction p ≤ 0.05). Visualisation of allele frequencies We visualised allele frequencies of amino acid substitutions in form of a heatmap. Pre-processed VCF files were annotated using SnpEff [54] (10.4161%2Ff) with the manually added lyrata v.2 reference annotation [55] (10.1371/journa). Variants annotated as missense (i.e. amino acid substitutions) were extracted using SnpSift [54] . Gene-coding loci were extracted from the whole-genome annotated VCF and per-population allele frequencies for each amino acid substitution calculated using GATK’s SelectVariants. Alternative allele frequencies (polarised against the lyrata reference) were visualised using the heatmap.2 function in the gplots package in R (Warnes et al., 2016, https://CRAN.R-project.org/pac ). Identification of differentiated and introgressed regions To investigate how the relationships among diploid and tetraploid populations of the two species vary across the genome, we used topology weighting by iterative sampling of subtrees ( Twisst ) [40] [ www.github.com/simonhmartin/twisst/ ]. Twisst provides a quantitative measure of the relationships among a set of taxa when each taxon is represented by multiple individuals and the taxa are not necessarily reciprocally monophyletic. This provides a naive means to detect both introgression and ILS, and how these vary across the genome. We first inferred genealogies for 50 SNP windows across the whole genome using the BIONJ algorithm [56] as implemented in PHYML [57] . As each individual carries two (for diploids) or four (for tetraploids) distinct haplotypes that represent different tips in the genealogy, it is necessary to first separate the haplotypes by phasing heterozygous genotypes. We used a heuristic approach to estimate phase that maximises the average extent of LD among all pairs of polymorphic sites in the window. This approach iteratively selects the best genotype configuration for each site, beginning with the site that has the most heterozygous genotypes. At each step, the optimal configuration is that which maximises the average LD between the target site and all previous target sites. This allows simultaneous phasing of diploids and tetraploids. We investigated the accuracy of this phasing approach using simulated sequences generated using the coalescent simulator msms [58] and seq-gen [59] , following [40] , but here adding steps to randomise phase and then apply phase inference. As Twisst is robust to within-taxon phasing errors [40] , the relevant question here is the extent to which imperfect phasing would affect the estimated topology weightings. We therefore applied Twisst to the simulated data and compared the results with (i) perfect phase, (ii) randomised phase and (iii) randomised and then inferred phase. This confirmed that our heuristic phasing algorithm led to an improvement in the accuracy of the weightings, giving results that approached what is achieved with perfect phase information. For running Twisst on the empirical data, we combined samples into four ingroup populations: diploid lyrata , tetraploid lyrata , diploid arenosa and tetraploid arenosa , and included A. halleri as outgroup. These five taxa give fifteen possible rooted taxon topologies (Fig. 3a ). Although Twisst does not consider rooting when computing topology weightings, the inclusion of an outgroup improves the interpretation of the results, allowing the direction of introgression to be inferred in some cases [40] . In all analyses, topology weightings were computed exactly for all window trees that could be simplified to ≤2,000 remaining haplotype combinations (see ref. [40] for details). In cases where this was not possible, approximate weightings were computed by randomly sampling combinations of haplotypes until the 95% binomial confidence interval for all fifteen topology weightings was below 0.05. Confidence intervals were computed using the Wilson method implemented in the package binom in R (R Core Team 2015). Reporting summary Further information on research design is available in the Nature Research Reporting Summary linked to this article.